Light helicity detector based on 2D magnetic semiconductor CrI3 Two-dimensional magnetic semiconductors provide a platform for studying physical phenomena at atomically thin limit, and promise magneto-optoelectronic devices application. Here, we report light helicity detectors based on graphene-CrI 3 -graphene vdW heterostructures. We investigate the circularly polarized light excited current and reflective magnetic circular dichroism (RMCD) under various magnetic fields in both monolayer and multilayer CrI 3 devices. The devices exhibit clear helicity-selective photoresponse behavior determined by the magnetic state of CrI 3 . We also find abnormal negative photocurrents at higher bias in both monolayer and multilayer CrI 3 . A possible explanation is proposed for this phenomenon. Our work reveals the interplay between magnetic and optoelectronic properties in CrI 3 and paves the way to developing spin-optoelectronic devices. Since the first discovery of intrinsic ferromagnetism in two-dimensional (2D) van der Waals (vdW) crystals of Cr 2 Ge 2 Te 6 and CrI 3 in 2017 [1] , [2] , 2D magnetic materials have aroused wide research interest. They provide a platform for studying light–matter interactions and magneto-optical/electrical phenomena at the atomically thin limit and also promise magneto-optoelectronic devices application [3] . Monolayer CrI 3 has ferromagnetic (FM) nature, whereas multilayer CrI 3 has a layered antiferromagnetic (AFM) nature with an easy magnetization axis perpendicular to the layers [2] , [4] , [5] , [6] . To date, various studies about CrI 3 were reported, including helical luminescence [7] , tunneling magnetoresistance [5] , [6] , [8] and electrostatic doping [9] , which demonstrated that the optical/electrical properties of CrI 3 are coupled with its magnetic property. To further study 2D magnetic semiconductor materials and advance their application, understanding the interplay between their magnetic and optoelectronic properties and developing magneto-optoelectronic devices are indispensable. In this work, we fabricate light helicity detectors based on graphene-CrI 3 -graphene vdW heterostructures and study their helical photoresponse properties via magneto-optoelectronic measurements. Devices with two representative thicknesses (monolayer and multilayer) of CrI 3 are investigated. We investigate their circularly polarized light excited current and reflective magnetic circular dichroism (RMCD) under various magnetic fields μ 0 H and temperatures. The devices exhibit helicity-selective photoresponse behavior determined by the magnetic state of CrI 3 . Both the helicity-dependent photocurrent and illumination-dependent tunneling current are studied in detail. The calculated photoresponsivity polarization has a clear relation with magnetic field, consistent with the RMCD signals. For the monolayer CrI 3 device, when the applied magnetic field switches the CrI 3 between the up magnetized state ( μ 0 H > 0.1 T) and the down magnetized state ( μ 0 H < −0.1 T), the photoresponsivity polarization ( \(\rho\) ) changes between ~−6 and +6%, and the RMCD signal changes between ~+1 and −1%. The photoresponsivity polarization equals zero, i.e., the helicity-dependent photoresponse phenomenon vanishes, at temperature higher than 40 K, close to the Curie temperature ( T c ) of monolayer CrI 3 (45 K) [2] . For the multilayer (14 nm thick) CrI 3 device, \(\rho\) value displays multiple plateaus with magnetic field sweeping, and saturates at ~±4.5% when | μ 0 H | > 2.2 T, corresponding to different spin configurations in CrI 3 enabled by spin-flip transitions at different magnetic fields. Specifically, for both monolayer and multilayer CrI 3 devices, the light-on current decreases with increasing excitation power at a higher bias. Based on detailed discussions, we provide a possible explanation to this phenomenon. Our work reveals the interplay between magnetic and optoelectronic properties in CrI 3 , and paves the way to developing spin-optoelectronic devices. Device fabrication and characterization The CrI 3 based light helicity detector was fabricated by mechanically exfoliating and dry transferring few-layer graphene, CrI 3 , and hexagonal boron nitride ( h BN) flakes from their bulk crystals to construct graphene-CrI 3 -graphene heterostructure. To avoid degradation [8] , the device was encapsulated by h BN flakes. The top and bottom graphene layers act as the electrodes. All the procedures were conducted in a glove box within an inert atmosphere (<0.1 ppm of water and oxygen) (see Methods). 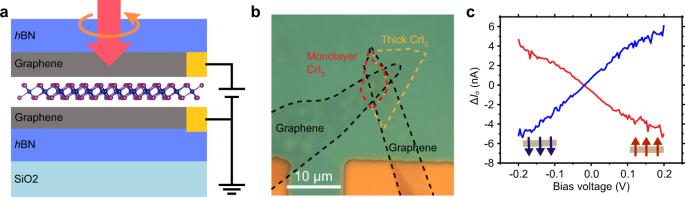Fig. 1: The monolayer CrI3light helicity detector D1. Schematic diagram (a) and optical micrograph (b) of a monolayer CrI3(demarcated by the red dashed lines) light helicity detector D1 with few-layer graphene contacts (demarcated by the black dashed lines). The yellow dashed lines demarcate the thick CrI3, which was not illuminated by the excitation light in the measurements. The device is encapsulated byhBN flakes.cThe difference of the light-on currents (ΔIσ=I+−I−) under\({\sigma }^{+}\)and\({\sigma }^{-}\)excitations as function of the bias, measured atμ0H= 0 T. Before being measured, the monolayer CrI3device was fully magnetized at |μ0H| > 0.3 T. The red (blue) color denotes up (down) magnetized CrI3. The ΔIσ–Vcurve shows negative (positive) slope for up (down) magnetized state of monolayer CrI3. These results show that the photocurrents in a fully magnetized CrI3is helicity-dependent. Figure 1a, b show the schematic diagram and optical image, respectively, of a monolayer CrI 3 light helicity detector D1. We measured the circularly polarized light excited current and RMCD of the device under various magnetic fields and temperatures. Both the excitation light and magnetic field μ 0 H are perpendicular to the 2D layers and parallel to the easy magnetization axis of CrI 3 (see Methods). Notably, in the experiment, the beam diameter of the excitation light is about 1 μm, less than the scale of vertical tunneling junction. For photoresponse and RMCD measurements, the temperature is 2 K and the excitation power is 10 μW, unless otherwise specified. Fig. 1: The monolayer CrI 3 light helicity detector D1. Schematic diagram ( a ) and optical micrograph ( b ) of a monolayer CrI 3 (demarcated by the red dashed lines) light helicity detector D1 with few-layer graphene contacts (demarcated by the black dashed lines). The yellow dashed lines demarcate the thick CrI 3 , which was not illuminated by the excitation light in the measurements. The device is encapsulated by h BN flakes. c The difference of the light-on currents (Δ I σ = I + − I − ) under \({\sigma }^{+}\) and \({\sigma }^{-}\) excitations as function of the bias, measured at μ 0 H = 0 T. Before being measured, the monolayer CrI 3 device was fully magnetized at | μ 0 H | > 0.3 T. The red (blue) color denotes up (down) magnetized CrI 3 . The Δ I σ – V curve shows negative (positive) slope for up (down) magnetized state of monolayer CrI 3 . These results show that the photocurrents in a fully magnetized CrI 3 is helicity-dependent. Full size image Circularly excited light-on currents The monolayer CrI 3 device was first fully magnetized at | μ 0 H | > 0.3 T. Then its light-on currents ( I light ) were measured at μ 0 H = 0 T under both right circularly polarized light ( \({\sigma }^{+}\) ) and left one ( \({\sigma }^{-}\) ) excitations. Their difference (Δ I σ = I + − I − ) is plotted as a function of applied bias ( V ) in Fig. 1c , where \({I}_{\pm }\) are the light-on currents under \({\sigma }^{\pm }\) excitations. The Δ I σ – V curves exhibit distinguishable difference between the I light under \({\sigma }^{+}\) and \({\sigma }^{-}\) excitations, with negative (positive) slope for the up (down) magnetized state of monolayer CrI 3 . These results show that the photocurrent in a fully magnetized CrI 3 is helicity-dependent. Light Power dependent magneto-optoelectronic response The excitation power dependent current versus bias relations ( I – V curves) of a monolayer CrI 3 with down magnetized state under \({\sigma }^{+}\) excitation at μ 0 H = 0 T (increased from –0.3 T) are shown in Fig. 2a . For identical bias, the I light increases monotonically with the excitation power. We calculate photoresponsivity \(R=\frac{{I}_{{{{{{\rm{ph}}}}}}}}{P}\) , where I ph is the photocurrent defined as I ph = I light – I dark , I dark is dark current (i.e., tunneling current in dark), and P is the excitation power. 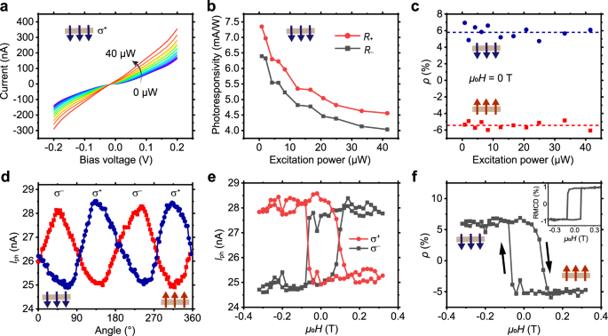Fig. 2: The magneto-optoelectronic response in the monolayer CrI3device D1. aI–Vcurves of the device with a down magnetized state under\({\sigma }^{+}\)excitation with various powers (from 0 to 40 μW) measured atμ0H= 0 T (increased from −0.3 T). For identical bias, the light-on current (Ilight) increases monotonically with the excitation power.bExcitation power-dependent photoresponsivities (R+andR−) measured atV= 0.2 V under\({\sigma }^{+}\)(red) and\({\sigma }^{-}\)(black) excitations in the down magnetized state CrI3.cExcitation power dependent photoresponsivity polarization\(\rho\)measured atμ0H= 0 T. The\(\rho\)is independent of excitation power with average values of ~−6% (red dashed line) for the up state (red dots) and ~+6% (blue dashed line) for the down state (blue dots).dPhotocurrents, measured atV= 0.15 V, versus the angle of the quarter-wave plate. The up (down) state CrI3exhibits a higher\({\sigma }^{-}\)(\({\sigma }^{+}\)) photocurrent.eCircularly excited photocurrents under various magnetic fields. The red (black) color denotes the\({\sigma }^{+}\)(\({\sigma }^{-}\)) excitation result. Whenμ0Hsweeps between ±0.3 T, the photocurrent behaviors are opposite for\({\sigma }^{+}\)and\({\sigma }^{-}\)excitation.fThe photoresponsivity polarization\(\rho\)values and the reflective magnetic circular dichroism (RMCD) signals (the inset) at variousμ0H. Whenμ0Hsweeps between −0.3 and +0.3 T,\(\rho\)changes between 6 and −6%, and RMCD signal changes between −1 and +1%. The CrI3spin-flip transitions occur at ±0.1 T. The excitation power dependent R + (under \({\sigma }^{+}\) excitation) and R − (under \({\sigma }^{-}\) excitation) at V = 0.2 V are plotted in Fig. 2b . The clear difference between the R + and R − illustrates again that the photocurrent is helicity-dependent and the device can serve as a light helicity detector [10] . The key parameter for a helicity detector is the photoresponsivity polarization defined as \(\rho =\frac{{R}_{+}-{R}_{-}}{{R}_{+}+{R}_{-}}\) , where \({R}_{\pm }\) are the \({\sigma }^{\pm }\) photoresponsivities [11] . Based on the above results, we obtain \(\rho \approx -6\) % (6%) for the up (down) magnetized monolayer CrI 3 at μ 0 H = 0 T, which, represented by red (blue) dots in Fig. 2c , is independent of excitation power. Fig. 2: The magneto-optoelectronic response in the monolayer CrI 3 device D1. a I – V curves of the device with a down magnetized state under \({\sigma }^{+}\) excitation with various powers (from 0 to 40 μW) measured at μ 0 H = 0 T (increased from −0.3 T). For identical bias, the light-on current ( I light ) increases monotonically with the excitation power. b Excitation power-dependent photoresponsivities ( R + and R − ) measured at V = 0.2 V under \({\sigma }^{+}\) (red) and \({\sigma }^{-}\) (black) excitations in the down magnetized state CrI 3 . c Excitation power dependent photoresponsivity polarization \(\rho\) measured at μ 0 H = 0 T. The \(\rho\) is independent of excitation power with average values of ~−6% (red dashed line) for the up state (red dots) and ~+6% (blue dashed line) for the down state (blue dots). d Photocurrents, measured at V = 0.15 V, versus the angle of the quarter-wave plate. The up (down) state CrI 3 exhibits a higher \({\sigma }^{-}\) ( \({\sigma }^{+}\) ) photocurrent. e Circularly excited photocurrents under various magnetic fields. The red (black) color denotes the \({\sigma }^{+}\) ( \({\sigma }^{-}\) ) excitation result. When μ 0 H sweeps between ±0.3 T, the photocurrent behaviors are opposite for \({\sigma }^{+}\) and \({\sigma }^{-}\) excitation. f The photoresponsivity polarization \(\rho\) values and the reflective magnetic circular dichroism (RMCD) signals (the inset) at various μ 0 H . When μ 0 H sweeps between −0.3 and +0.3 T, \(\rho\) changes between 6 and −6%, and RMCD signal changes between −1 and +1%. The CrI 3 spin-flip transitions occur at ±0.1 T. Full size image Magnetic order dependence of the helical photocurrents In order to further investigate the relation between the helical photocurrent and the intrinsic magnetism of the monolayer CrI 3 , we directly measured the photocurrent I ph ( V = 0.15 V) of D1 under various magnetic fields μ 0 H by the lock-in technique. The excitation laser is modulated to switch between \({\sigma }^{+}\) and \({\sigma }^{-}\) by a quarter wave plate equipped with a motorized rotation stage (see Methods). The circularly polarized photocurrent versus the phase of the quarter-wave plate relations for upstate (red dots) and downstate CrI 3 (blue dots) are opposite (Fig. 2d ), with I ph ( \({\sigma }^{+}\) ) > I ph ( \({\sigma }^{-}\) ) for the down state CrI 3 , and vice versa. When μ 0 H sweeps between ±0.3 T, the photocurrent behaviors are opposite for \({\sigma }^{+}\) and \({\sigma }^{-}\) excitation as shown in Fig. 2e . By curve fitting the data as shown in Fig. 2d with a cosine function, we can obtain the corresponding photoresponsivity polarization \(\rho\) . When μ 0 H sweeps between −0.3 and 0.3 T, \(\rho\) changes between 6 and −6% (Fig. 2f ), correspondingly, the RMCD signal changes between −1 and +1% (the inset in Fig. 2f ). The monolayer CrI 3 spin-flip transitions occur at ±0.1 T. While the device exhibits significant magnetic field-dependent helical photocurrent property, the dark tunneling current I dark is almost independent of the magnetic field as shown in Supplementary Fig. 1 , because the resistances of the down- or up-magnetized CrI 3 are equal. All the above results demonstrate that the magnetic field-dependent circularly polarized photocurrent can be used to detect the helicity of the incident light. We also measured the photoresponsivity polarization \(\rho\) of the helicity detector D1 under the zero-field-cooling condition (Fig. 3 ). When the temperature decreases from 80 to 2 K, \(\rho\) increases from 0% to a saturation value of 6% (black dots). By curve fitting the data with \(\rho \left(T\right)={\rho }_{0}{(1-\frac{T}{{T}_{c}})}^{\beta }\) (red line), where \({\rho }_{0}\) is the critical amplitude, \(\beta\) is the critical exponent, we obtain T c = 40 K, close to the Curie temperature of monolayer CrI 3 (45 K). Fig. 3: Temperature-dependent photoresponsivity polarization of the light helicity detector D1 measured at zero magnetic field. As temperature decreases from 80 to 2 K, \(\rho\) (black dots) increases from 0% (the dashed line) to a saturated value of 6%, corresponding to the down magnetized state of CrI 3 . The helicities \(\rho\) , together with the error bars, are obtained by fitting the relation between the photocurrent and the angle of the quarter-wave plate. By fitting the data with \(\rho \left(T\right)={\rho }_{0}{(1-\frac{T}{{T}_{{{{{{\rm{c}}}}}}}})}^{\beta }\) (red line), we obtain T c = 40 K. Full size image The origin of the helicity-dependent photocurrent can be understood by analyzing the split energy band structure in a fully magnetized CrI 3 [12] , [13] as shown in Supplementary Fig. 2a . The energy bands for electrons with different spins exhibit different band gaps. The narrower band gap corresponds to majority-spin electrons, and vice versa. Under the 633 nm light excitation, only the majority-spin electrons can be excited and form a few types of excitons [7] , [14] . 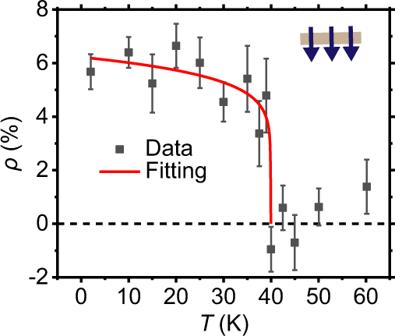Fig. 3: Temperature-dependent photoresponsivity polarization of the light helicity detector D1 measured at zero magnetic field. As temperature decreases from 80 to 2 K,\(\rho\)(black dots) increases from 0% (the dashed line) to a saturated value of 6%, corresponding to the down magnetized state of CrI3. The helicities\(\rho\), together with the error bars, are obtained by fitting the relation between the photocurrent and the angle of the quarter-wave plate. By fitting the data with\(\rho \left(T\right)={\rho }_{0}{(1-\frac{T}{{T}_{{{{{{\rm{c}}}}}}}})}^{\beta }\)(red line), we obtainTc= 40 K. These excitons obey the helicity-selective transition rule (Supplementary Fig. 2b ), determined by the optical selection rules. From the frequency-dependent circularly polarized absorbance of ferromagnetic monolayer CrI 3 at normal incidence [14] , we can see that, at the 633 nm (1.96 eV) excitation wavelength, \({\sigma }^{+}\) and \({\sigma }^{-}\) light absorbances are different, which are dominated by the B + and B − bright exciton absorbances, respectively, leading to the helicity-dependent photocurrent under applied bias. The helicity-dependent absorption is also demonstrated by the RMCD signals (the inset in Fig. 2f ), which indicate the difference in reflectivity of the \({\sigma }^{+}\) and \({\sigma }^{-}\) light (see Methods). 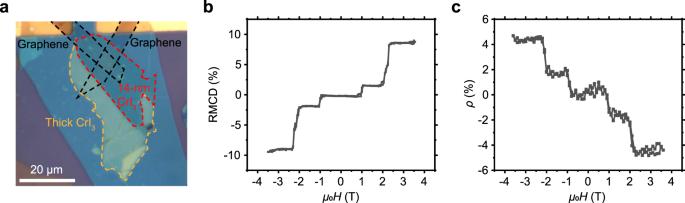Fig. 4: The multilayer CrI3light helicity detector D2. aOptical image of the 14 nm thick CrI3(demarcated by the red dashed lines) light helicity detector D2 with few-layer graphene contacts (demarcated by the black dashed lines). The yellow dashed lines demarcate the thick CrI3, which was not illuminated by the excitation light in the measurements. The device is encapsulated byhBN flakes. The reflective magnetic circular dichroism (RMCD) signals (b) and photoresponsivity polarization\(\rho\)(c) versusμ0Hrelations of the device. Both RMCD and\(\rho\)show five plateaus whenμ0Hsweeps between −3.5 and +3.5 T, and equal 0 atμ0H= 0 T, corresponding to the AFM ground state. RMCD signals and\(\rho\)values saturate at ~±10 and ±4.5%, respectively, when |μ0H| > 2.2 T, corresponding to the fully spin-polarized states. 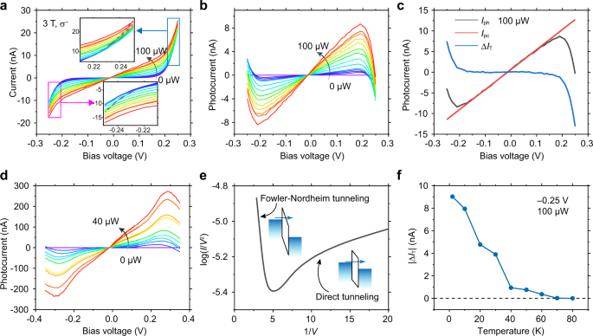Fig. 5: The abnormal negative photocurrent in the CrI3devices. aI–Vcurves of the ~10 nm thick CrI3light helicity detector D3 under\({\sigma }^{-}\)excitation with various powers (from 0 to 100 μW) atμ0H= 3 T. The insets: the zoomed-in regions at higher bias. TheIlight–Vcurves are linear withinV= ±0.19 V, but become nonlinear and cross to each other at higher bias.bThe photocurrentsIphobtained from (a) by subtractingIdarkfromIlight. For all the excitation powers, theIphincreases linearly with bias within ±0.19 V, but deviates from linear behavior and even decreases at higher bias, resulting in a negative photocurrent.cTheIph–Vcurve under 100 μW excitation (black line), theIpc–Vcurve extracted by linear fitting theIph–Vcurve withinV= ±0.15 V, and extending the result to the full bias range of ±0.25 V (red line), and the ΔIT–Vcurve (blue line) obtained by subtractingIpcfromIph. Under light illumination, the tunneling current decreases for bias voltages |V| > 0.19 V.dTheIph–Vcurves in the monolayer CrI3device D1 under various excitation powers atμ0H= 0 T. The negative photocurrent phenomenon occurs at bias higher than 0.25 V.eThe dark tunneling currents in the monolayer CrI3device D1 are plotted in the log(I/V2)–1/Vdiagram. The negative (positive) slope of the curve at high (low) bias region indicates the Fowler–Nordheim tunneling (direct tunneling) mechanism. The two insets: the energy band diagrams of the two tunneling mechanism, the left for the Fowler–Nordheim tunneling and the right for the direct tunneling.fThe temperature-dependent | ΔIT| in D3 measured atV= −0.25 V under 100 μW light excitation. With the temperature increasing, |ΔIT| decreases monotonously until zero (the dashed line) at a temperature higher than 60 K. Helical photocurrents in multilayer CrI 3 helicity detector Figure 4a shows an optical image of a 14 nm thick CrI 3 light helicity detector D2. The magnetoresistances measured in dark at V = 0.3 V under various magnetic fields are shown in Supplementary Fig. 3a . The magnetoresistance is significant with abrupt changes around ±1 and ±2 T, consistent with the RMCD result (Fig. 4b ). The I dark − V curves at three representative magnetic field (0, 1.5, and 3 T) are shown in Supplementary Fig. 3b . We can see that, for the applied magnetic fields in our experiment, the tunneling currents in dark are negligible within V = ±0.19 V. To eliminate the influence of the tunneling current (to be discussed in the next section), herein, the photocurrents are measured at V = −0.15 V under various magnetic fields by the lock-in technique. Both the RMCD signal (Fig. 4b ) and photoresponsivity polarization \(\rho\) (Fig. 4c ) show five plateaus when μ 0 H sweeps between −3.5 and +3.5 T, corresponding to five magnetic states enabled by the layered AFM nature of multilayer CrI 3 . The photoresponsivity polarization \(\rho\) equals 0 at μ 0 H = 0 T, corresponding to the AFM ground state, and saturates at ±4.5% when | μ 0 H | > 2.2 T, corresponding to the fully spin-polarized states. Fig. 4: The multilayer CrI 3 light helicity detector D2. a Optical image of the 14 nm thick CrI 3 (demarcated by the red dashed lines) light helicity detector D2 with few-layer graphene contacts (demarcated by the black dashed lines). The yellow dashed lines demarcate the thick CrI 3 , which was not illuminated by the excitation light in the measurements. The device is encapsulated by h BN flakes. The reflective magnetic circular dichroism (RMCD) signals ( b ) and photoresponsivity polarization \(\rho\) ( c ) versus μ 0 H relations of the device. Both RMCD and \(\rho\) show five plateaus when μ 0 H sweeps between −3.5 and +3.5 T, and equal 0 at μ 0 H = 0 T, corresponding to the AFM ground state. RMCD signals and \(\rho\) values saturate at ~±10 and ±4.5%, respectively, when | μ 0 H | > 2.2 T, corresponding to the fully spin-polarized states. Full size image The abnormal negative photocurrents at higher bias The I – V curves of a ~10 nm thick CrI 3 light helicity detector D3 are measured at μ 0 H = 3 T under \({\sigma }^{-}\) excitation with various powers (from 0 to 100 μW) (Fig. 5a ). The I – V curves are linear within V = ±0.19 V, but become nonlinear and cross to each other at higher biases (e.g., 0.25 V, the insets in Fig. 5a ). Specifically, for identical bias within ±0.19 V, the I light increases monotonically with the excitation power increasing. However, it decreases first and then increases with the excitation power increasing at a higher bias, e.g., V = 0.25 V (Supplementary Fig. 4 ). Such intriguing phenomenon can be reproduced in D2 (Supplementary Fig. 5 ). We extract the photocurrents I ph by subtracting I dark from I light (Fig. 5a ) as shown in Fig. 5b . We can see that, for all the excitation powers, I ph increases linearly with bias within V = ±0.19 V, but deviates from linear behavior and even decreases at higher bias, resulting in a negative photocurrent. The critical biases of ±0.19 V coincide with the bias at which I dark becomes significant (see the 0 μW excited I – V curve in Fig. 5a ). Fig. 5: The abnormal negative photocurrent in the CrI 3 devices. a I – V curves of the ~10 nm thick CrI 3 light helicity detector D3 under \({\sigma }^{-}\) excitation with various powers (from 0 to 100 μW) at μ 0 H = 3 T. The insets: the zoomed-in regions at higher bias. The I light – V curves are linear within V = ±0.19 V, but become nonlinear and cross to each other at higher bias. b The photocurrents I ph obtained from ( a ) by subtracting I dark from I light . For all the excitation powers, the I ph increases linearly with bias within ±0.19 V, but deviates from linear behavior and even decreases at higher bias, resulting in a negative photocurrent. c The I ph – V curve under 100 μW excitation (black line), the I pc – V curve extracted by linear fitting the I ph – V curve within V = ±0.15 V, and extending the result to the full bias range of ±0.25 V (red line), and the Δ I T – V curve (blue line) obtained by subtracting I pc from I ph . Under light illumination, the tunneling current decreases for bias voltages | V | > 0.19 V. d The I ph – V curves in the monolayer CrI 3 device D1 under various excitation powers at μ 0 H = 0 T. The negative photocurrent phenomenon occurs at bias higher than 0.25 V. e The dark tunneling currents in the monolayer CrI 3 device D1 are plotted in the log( I / V 2 )–1/ V diagram. The negative (positive) slope of the curve at high (low) bias region indicates the Fowler–Nordheim tunneling (direct tunneling) mechanism. The two insets: the energy band diagrams of the two tunneling mechanism, the left for the Fowler–Nordheim tunneling and the right for the direct tunneling. f The temperature-dependent | Δ I T | in D3 measured at V = −0.25 V under 100 μW light excitation. With the temperature increasing, |Δ I T | decreases monotonously until zero (the dashed line) at a temperature higher than 60 K. Full size image In order to explore the abnormal negative photocurrent phenomenon in multilayer CrI 3 devices, we consider that the I light includes the photocurrent I ph and the tunneling current in dark I dark . The I ph includes the photoconductive current I pc and the variation of the tunneling current under light illumination Δ I T . Given a linear relationship between the I pc and applied bias V , we extract the photoconductivity current I pc by linear fitting the I ph – V curve (under 100 μW excitation) within V = ±0.15 V, and extending the result to the full bias range of ±0.25 V (red line in Fig. 5c ). Next, we obtain the Δ I T (blue line in Fig. 5c ) by subtracting I pc (red line) from the photocurrent I ph (black line). We can see that, under light illumination, the tunneling current reduces at a higher bias (| V | > 0.19 V), and the reduction magnitude | Δ I T | increases monotonically with excitation power (Supplementary Fig. 6 ). If normalize the Δ I T – V and I dark – V curves by their respective current values at V = 0.25 V, we find that the two curves overlap well with each other (Supplementary Fig. 7 ), indicating that the Δ I T is proportional to the I dark , regardless of the applied bias. These results suggest that the abnormal negative photocurrent phenomenon at higher bias in multilayer CrI 3 devices may result from tunneling current reduction under light illumination. It is worth noting that the negative photocurrent phenomenon can also be observed in the monolayer CrI 3 device at a higher bias (| V | > 0.25 V, Fig. 5d ). We plot the dark tunneling current in a log( I / V 2 ) vs. 1/ V diagram [15] , [16] to examine the tunneling mechanisms in both monolayer and multilayer CrI 3 . The log( I / V 2 )−1/ V curve for monolayer device (Fig. 5e ) shows negative (positive) slope at higher (lower) bias region, corresponding to Fowler–Nordheim (FN) tunneling (direct tunneling) [17] . Direct tunneling occurs in the lower bias region, i.e., the carriers directly tunnel through a trapezoidal barrier (the right inset in Fig. 5e ) without entering into the conduction band of semiconductor [18] . FN tunneling occurs in a higher bias region (>0.25 V for monolayer CrI 3 case), wherein the energy band bends more and the electrons tunnel into the conduction band of the semiconductor (the left inset in Fig. 5e ) [6] , [8] . The log( I / V 2)−1/ V curve for the ~10-nm CrI 3 device D3 is shown in Supplementary Fig. 8 , where the FN tunneling occurs at V > 0.19 V. These results indicate that there exists a relationship between the abnormal photocurrent and the tunneling current with FN tunneling mechanism. We further perform the temperature-dependent measurement in the ~10 nm thick CrI 3 device D3. As temperature increases, the | Δ I T | (measured at V = −0.25 V) exhibits a monotonous decrease until zero at a temperature higher than the Curie temperature of CrI 3 ( T c = 61 K [4] ). This result indicates that the negative photocurrent phenomenon weakens as temperature increases, and vanishes at temperature higher than 60 K. The temperature dependence of the dark tunneling current I dark for the 10-nm CrI 3 device is shown in Supplementary Fig. 9a . As the temperature increases from 2 K, the I dark first decreases and then increases. The turning point is 60 K. Similar result was reported previously for CrI 3 tunneling device [8] . The I ph − V relations at various temperatures are shown in Supplementary Fig. 9b . At lower temperature, the I ph − V curves are nonlinear due to the negative photocurrent. As temperature increases, the I ph − V curves become linear, corresponding to the weakening negative photocurrent phenomenon. One possible origin for the abnormal negative photocurrent phenomenon is the light-induced defects in CrI 3 [19] . The defects may trap the electrons which tunnel into the conduction band of CrI 3 through FN tunneling, resulting in reduced conductivity. At higher temperatures ( k B T > activation energy of the trapped electron), the trapped electrons would release and contribute again to conductivity. Therefore, the absolute value of Δ I T decreases with increasing temperature as shown in Fig. 5f . Nevertheless, to fully verify this, further study of dynamic process of the interaction between photons and electrons is needed. In conclusion, we fabricated light helicity detectors based on graphene-CrI 3 -graphene vdW heterostructures and measured their circularly polarized light excited current and RMCD under various magnetic fields. The helicity-dependent photocurrent has a clear relation with a magnetic field, consistent with the RMCD result. For the monolayer CrI 3 device D1, the photoresponsivity polarization switches between ±6% as the magnetic field sweeps between ±0.3 T. The helicity-dependent photoresponse phenomenon vanishes at temperature higher than 40 K, close to the Curie temperature ( T c ) of monolayer CrI 3 (45 K). For the multilayer CrI 3 device, the photoresponsivity polarization performs AFM properties that saturates at ±4.5% when | μ 0 H | > 2.2 T, and equals 0 at μ 0 H = 0 T. Moreover, we find abnormal negative photocurrent phenomenon at higher bias in both monolayer and multilayer CrI 3 . We try to unveil the origin of this phenomenon by investigating the tunneling current mechanism in CrI 3 , together with the temperature dependent measurement. Our work reveals the interplay between magnetic and optoelectronic properties in CrI 3 and paves the way to developing spin-optoelectronic devices. Device fabrication First, few-layer graphene, CrI 3 , and h BN (10–30 nm) flakes were exfoliated onto polydimethylsiloxane (PDMS) substrates in an argon gas-filled glove box with <0.1 ppm concentration of oxygen and water. Then, the h BN encapsulated graphene-CrI 3 -graphene heterostructure was assembled layer-by-layer on a Si/SiO 2 substrate in the same glove box with the dry transferring method using the PDMS substrate as stamp under the help of a microscope attached with a micro-manipulator. The two graphene electrodes were contacted to the pre-prepared Cr/Au (5/25 nm) electrodes for measuring purpose. The thicknesses of the flakes were estimated by optical contrast and confirmed by atomic force microscopy after device measurements. RMCD and magneto-optoelectronic measurements Both RMCD and magneto-optoelectronic measurements were performed in a dry cryostat (attoDRY2100, base temperature of 1.7 K) equipped with a 9 T superconducting magnet and a home tailored microscopic setup in back-scattering geometry. The RMCD is defined as \(({R}_{\sigma +}-{R}_{\sigma -})/({R}_{\sigma +}+{R}_{\sigma -})\) , where \({R}_{\sigma \pm }\) are the intensities of the \({\sigma }_{\pm }\) reflected light. For RMCD measurement, the temperature was 2 K, and the device was illuminated by a 633 nm He-Ne laser with a power of 10 μW. The laser was modulated by a chopper and a photoelastic modulator (PEM100), and was focused on the device with a beam diameter ~1 μm by a low-temperature apochromatic objective (LT-APO/VISIR/0.82). The collected light from the sample via the same objective was sent to a photomultiplier tube (PMT1001) equipped with a lock-in amplifier (HF2LI). For magneto-optoelectronic measurement, circularly polarized light was realized by modulating the 633 nm He-Ne laser with a polarizer and a quarter wave plate equipped with a motorized rotation stage. A chopper was employed to switch the light between on and off states with a frequency of 73 Hz. The photocurrent was measured directly by the lock-in amplifier. The I – V curves were measured with a Keithley 2636B source/measure unit. The temperature was 2 K and the excitation power was 10 μW, unless otherwise specified.